Aging mechanisms in amorphous phase-change materials Aging is a ubiquitous phenomenon in glasses. In the case of phase-change materials, it leads to a drift in the electrical resistance, which hinders the development of ultrahigh density storage devices. Here we elucidate the aging process in amorphous GeTe, a prototypical phase-change material, by advanced numerical simulations, photothermal deflection spectroscopy and impedance spectroscopy experiments. We show that aging is accompanied by a progressive change of the local chemical order towards the crystalline one. Yet, the glass evolves towards a covalent amorphous network with increasing Peierls distortion, whose structural and electronic properties drift away from those of the resonantly bonded crystal. This behaviour sets phase-change materials apart from conventional glass-forming systems, which display the same local structure and bonding in both phases. Amorphous materials are out of thermodynamic equilibrium and, as such, are prone to temporal evolution. This phenomenon is called physical aging and is usually attributed to structural relaxation towards the equilibrium state [1] . Aging is ubiquitous in glasses and often detrimental for applications. It can result in a temporal drift of technologically important properties, such as the permeability of polymer glasses [2] , [3] or the electrical and optical properties of hydrogenated amorphous silicon employed in photovoltaic devices [4] . The amorphous state of so-called phase-change materials (PCMs) also exhibits aging. PCMs are used as the active part of non-volatile memory devices [5] , [6] , which exploit the fast and reversible switch between a conductive crystalline structure and an amorphous phase that displays a higher electrical resistivity. On aging, the resistivity of the amorphous state for a large number of such systems [7] , [8] , [9] increases even further. This ‘resistance drift’ impedes the realization of multilevel memories. It is therefore crucial to understand and eliminate this phenomenon to further boost the storage capabilities of phase-change memories. In principle, computer simulation is the method of choice to investigate such relaxation processes at the microscopic level. However, the complexity of the chemistry of these alloys requires accurate quantum-based density functional theory (DFT) calculations to properly describe and understand the bonding mechanisms in the amorphous phase. A second problem stems from the time scales involved in (a) the formation of the glass by quenching and in (b) aging at room temperature, which are both much longer than those accessible to direct DFT-based molecular dynamics simulations of the process. Since Zachariasen wrote his seminal paper [10] on the atomic arrangement in oxide glasses, it is common knowledge that the atoms in such glasses are linked together by forces that are essentially the same as those in crystals. Hence, the short-range order in oxide glasses closely resembles the atomic structure of the corresponding crystals. By contrast, PCMs along the GeTe-Sb 2 Te 3 line show significant differences in atomic arrangement between the amorphous and crystalline state [11] . This can be attributed to a pronounced difference in chemical bonding between the two phases, which is observed in all PCMs, including doped Sb 2 Te compounds, such as Ag- In-doped Sb2Te [12] , [13] . By now, it is reasonably well understood that the atomic structure of the crystalline phase is stabilized by resonant bonding, which is responsible for the high electronic polarisabilities and optical dielectric constants displayed by crystalline PCMs. Since this resonance effect requires long-range order [14] , [15] , it vanishes in amorphous PCMs, which instead exhibit ordinary covalent bonds [16] , [17] and correspondingly lower polarisabilities. This difference in bonding impedes the identification of the prevalent structural motif in amorphous PCMs based on knowledge of the corresponding crystalline phase. Indeed, for Ge x Sb y Te 1+ x + y alloys, DFT-based atomistic computer simulations [18] , [19] , [20] report a significant proportion of tetrahedrally bonded Ge atoms in the amorphous phase, while no crystalline phase with such Ge environment exists. These tetrahedrally coordinated Ge atoms, denoted Ge T , are obtained by quenching liquid configurations, thus mimicking the actual experimental process. Experimental cooling rates have to be very high to prevent crystallization (PCMs are poor glass formers [21] ); however, simulated quenches are even several orders of magnitude faster [22] , due to the computational cost of DFT-based molecular dynamics. This raises the question whether the tetrahedral structures observed in the DFT models are relevant to experiments or originate from the too high quench rates. In this paper, we address these issues by focusing on the prototype system GeTe. From the bonding and aging points of view this solid is representative of a wider class of PCMs located on the pseudobinary line between GeTe and Sb 2 Te 3 [23] , [24] , [25] . Our combined computational and experimental investigation elucidates the microscopic mechanisms responsible for aging in amorphous GeTe. We carry out simulations based on standard DFT functionals, as well as on non-local ‘van der Waals’ (vdW) functionals, to achieve the required accurate description of the atomic and electronic structure in the amorphous phase. To circumvent the time scale problem, we generate a collection of amorphous structures with various characteristic local bonding patterns, to explore the potential energy landscape relevant to aging. Then, using a new approximate technique to calculate the stability of these different local environments, we identify the driving forces leading to the resistivity drift, and assess our results by comparing computed characteristic properties with experimental photothermal deflection spectroscopy (PDS) data, as well as impedance spectroscopy data. Global stability of the amorphous network Our first goal is to clarify why DFT models of GeTe contain tetrahedral motifs. For this purpose, we perform melt-quench DFT simulations of three binary chalcogenides, namely GeSe, GeTe and SnTe. All of these compounds crystallize into a (distorted) rocksalt structure, characterized by an octahedral-like atomic arrangement. Nevertheless, for the Ge–Se system also a tetrahedrally bonded crystal phase exists, which has the stoichiometry GeSe 2 . No such phase exists for Ge–Te and Sn–Te. The inset of Fig. 1 displays the heats of formation [26] , [27] , [28] , [29] , [30] for octahedrally bonded IV–VI compounds like GeTe, as well as tetrahedrally bonded IV–VI 2 compounds like GeSe 2 . It can be clearly seen from the trends in the heat of formation that octahedral bonding is favoured for the heavier IV–VI compounds, like Ge–Te and Sn–Te, while tetrahedral bonding is favoured in the lighter alloys, such as GeS 2 . We use the second-generation Car–Parrinello method [31] , [32] , in combination with DFT and generalized gradient approximation (GGA) functionals [33] , to produce 10 amorphous models for each compound, starting from different liquid configurations. Our DFT results are shown in Fig. 1 . Amorphous SnTe contains almost no tetrahedral motifs. Remarkably, amorphous GeTe (a-GeTe) contains more tetrahedral Ge atoms (Ge T ) than a-GeSe. This finding is surprising at first sight, since one would have expected a higher number of tetrahedrally coordinated Ge atoms for the Ge–Se system, which can form a tetrahedrally bonded crystalline phase. However, our result can be understood by first noticing [20] , [34] that Ge T atoms are associated with the presence of homopolar Ge–Ge bonds. The heat of formation values for GeTe, GeSe and SnTe (see Fig. 1 inset) indicate that the formation of homopolar bonds in the molten state is easier in GeTe than in GeSe and SnTe. Due to the fast-quenching rate, the chemical order in the simulated amorphous state is similar to that in the liquid, which results in a large fraction of homopolar bonds and tetrahedral Ge T in a-GeTe. On average, the fractions of homopolar bonds in the liquid and amorphous states are about 18 and 12% for GeTe, against 7 and 1% for SnTe. 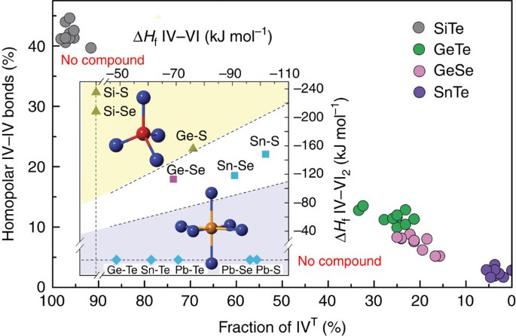Figure 1: Relation between homopolar ‘IV-IV bonds’ and tetrahedreal units. The fraction of homopolar ‘IV-IV bonds’ in amorphous IV–VI compounds (SiTe, GeTe, GeSe and SnTe) as a function of the fraction of tetrahedrally coordinated group IV atoms showing a close correlation. Inset: heat of formation of selected IV–VI (xaxis) and IV–VI2(yaxis) compounds. In the upper region, tetrahedral bonding is preferred, while octahedral bonding prevails in the lower part. The dashed line separates stable IV–VI and IV–VI2compounds, which feature preferential octahedral and tetrahedral bonding, respectively. The dotted lines mark those compounds, which do exist either only with an octahedral atomic arrangement with IV–VI stoichiometry (horizontal line), or only with a tetrahedral atomic arrangement with IV–VI2stoichiometry (vertical line). Figure 1: Relation between homopolar ‘IV-IV bonds’ and tetrahedreal units. The fraction of homopolar ‘IV-IV bonds’ in amorphous IV–VI compounds (SiTe, GeTe, GeSe and SnTe) as a function of the fraction of tetrahedrally coordinated group IV atoms showing a close correlation. Inset: heat of formation of selected IV–VI ( x axis) and IV–VI 2 ( y axis) compounds. In the upper region, tetrahedral bonding is preferred, while octahedral bonding prevails in the lower part. The dashed line separates stable IV–VI and IV–VI 2 compounds, which feature preferential octahedral and tetrahedral bonding, respectively. The dotted lines mark those compounds, which do exist either only with an octahedral atomic arrangement with IV–VI stoichiometry (horizontal line), or only with a tetrahedral atomic arrangement with IV–VI 2 stoichiometry (vertical line). Full size image Therefore, we have to prove whether these homopolar Ge bonds and tetrahedral Ge atoms are present in the relaxed glass as well. To shed light on this, we need a computational approach to produce amorphous GeTe, enabling us to ‘tune’ the fraction of Ge–Ge bonds. The similarity between the chemical orders of liquid and amorphous states generated by the fast DFT-molecular dynamics quenching and the Fig. 1 data indicate the way forward: to try to mimic the experimental melt-quench and aging process, we generate a number of a-GeTe structures by chemically substituting Sn by Ge in our models of amorphous SnTe, and replace Se by Te in a-GeSe. Furthermore, to create Ge T -rich amorphous GeTe, we also consider melt-quenched models of SiTe (wherein most Si atoms form homopolar bonds) and subsequently exchange Si by Ge. After substitution and relaxation, a-GeTe structures with variable fractions of homopolar bonds, almost linearly correlated with the fraction of tetrahedral Ge ( Fig. 2a ), are obtained. The dependence of the total energy on the fraction of Ge T atoms in the structures (relaxed at 0 K) is shown in Fig. 2a . Interestingly, this dependence is almost linear, the lowest energy structures corresponding to the smallest fraction of tetrahedral Ge and thus to the lowest proportion of homopolar bonds. Three atomic configurations corresponding to different energy levels are visualized in Fig. 2b–d . Notice that the tetrahedral-rich SiTe substituted models (b) exhibit phase separation. In principle, there could also exist amorphous networks of GeTe, where Ge atoms are tetrahedrally coordinated but no phase separation occurs (for example, networks consisting mainly of Ge T -[GeTe 3 ] structures). In our models, the average fraction of Ge T -[GeTe 3 ] is 14%. 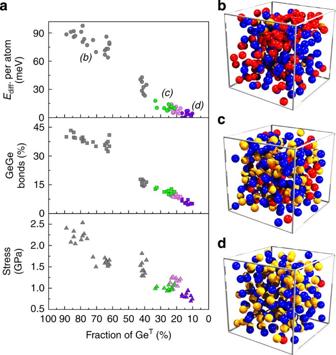Figure 2: Impact of tetrahedral environments on the global stability of amorphous GeTe. (a) Energy difference per atom, fraction of homopolar GeGe bonds, and stress of the relaxed models obtained by melt-quenching (green) and different chemical replacement procedures, substituting atoms from amorphous SnTe (violet), GeSe (light magenta) and SiTe (grey). (b–d) These panels correspond to different atomic configurations of amorphous GeTe in the energy difference plot. Te, tetrahedral Ge and defective octahedral Ge atoms are rendered with blue, red and orange spheres. The disappearance of tetrahedrally coordinated Ge atoms going from modelbtodis clearly discernible. Figure 2: Impact of tetrahedral environments on the global stability of amorphous GeTe. ( a ) Energy difference per atom, fraction of homopolar GeGe bonds, and stress of the relaxed models obtained by melt-quenching (green) and different chemical replacement procedures, substituting atoms from amorphous SnTe (violet), GeSe (light magenta) and SiTe (grey). ( b – d ) These panels correspond to different atomic configurations of amorphous GeTe in the energy difference plot. Te, tetrahedral Ge and defective octahedral Ge atoms are rendered with blue, red and orange spheres. The disappearance of tetrahedrally coordinated Ge atoms going from model b to d is clearly discernible. Full size image All the structures are generated at the density of amorphous GeTe (0.0334 Å −3 ), leading to internal stresses that follow the same linear behaviour as the energy ( Fig. 2a ), with Ge T -rich models exhibiting the largest values of stress. This implies that the presence of Ge T , and hence homopolar bonds, undermines the global stability of the network, since both terms of the enthalpy ( U + PV ) are minimized by the models displaying a small fraction of tetrahedral Ge. Homopolar bonds and Ge T atoms are thus kinetically stabilized by the fast-quenching rates but are energetically unfavourable. These findings suggest that the relaxation of the amorphous state and, by corollary, the drift process could be linked with the removal of homopolar bonds, in agreement with experiments showing [35] , [36] that the drift of PCMs is accompanied by stress relief. We show below that drift involves more than this, but we first have to understand why the removal of tetrahedrally coordinated Ge atoms reduces the energy and stress. For this purpose, we analyse the local bonding patterns in a-GeTe, which brings an additional challenge, because standard GGA functionals used in DFT tend to give too long first-neighbour distances. In ref. 37 , the semiempirical Grimme correction to DFT [38] was shown to reduce the deviations from experiments for Ge 15 Te 85 at high temperature. However, it fails to improve the agreement with experiments for amorphous GeTe (see Supplementary Note 1 and Supplementary Fig. 1 ). Here we employ the more complex vdW density functional proposed by Lee et al. [39] (denoted as vdW-DF2), which includes non-local correlations. We anneal the previously obtained GeTe structures using this functional, which does not modify the relative stability of the models, but leads to a better agreement with experimental data for the atomic arrangement (see Supplementary Figs 2 and 3 ). The new amorphous structures produced display atomic connectivities that are more sharply defined. Some Ge atoms are fourfold coordinated (Ge IV ) and are either tetrahedrally bonded, with four bonds around 109° (Ge T ), or form structures with four bonds closer to 90° (Ge H ), that are reminiscent of the high-pressure structure of Se or Te [40] . The remaining Ge atoms are threefold coordinated (denoted Ge III ) with three rigid bond angles around 90°. Both Ge III and Ge H structures result from a Peierls-like distortion of the octahedral first-neighbour shell of Ge. Te atoms are either two- or threefold coordinated (respectively, denoted Te II and Te III ) and mostly connected to Ge atoms. Local energy analysis To compare the relative stability of the local structures, one could follow the energy density approach that was shown to yield accurate defect and surface energies for crystals [41] . Instead, for our disordered systems, we develop an approximate method to calculate the contribution of each atom to the total energy of the system, by calculating the energy change upon removal of the selected atom from the structure, as explained in detail in the Supplementary Note 2 . The contribution of each Ge and Te atom to the total energy is displayed in Fig. 3 as a function of an order parameter denoted P i , which discriminates between the different local motifs (see Supplementary Note 3 , Supplementary Fig. 4 ). P i varies continuously from 1 (in Ge T , with 4 equal bonds, or Te III , with 3 equal bonds) to about 1.4 (for Ge III ) and 1.5 (for Te II ). In Fig. 3 we also plot the atomic volume distributions, obtained by a Voronoï tessellation analysis [42] . Both energies and volumes depend strongly on the bonding and chemical environment of the atom: fluctuations are thus large. Nevertheless, important information can be reliably obtained. We first see that tetrahedral Ge T (1.0≤ P Ge ≤1.10) are generally associated with twofold coordinated Te II (1.25≤ P Te ≤1.50), as seen most easily in the structures derived from SiTe (black symbols) containing a large number of homopolar bonds. Conversely, Te III (1.00≤ P Te ≤1.15) are dominant in SnTe-derived amorphous models (blue symbols), and are associated with Ge H and Ge III (1.15≤ P Ge ≤1.40). The local energy distributions for Ge and Te atoms behave very differently. Ge T ( E ≈−3.5 eV) and Ge III ( E ≈−3.7 eV) are almost degenerate, the latter being slightly favoured, whereas intermediate Ge H (1.10≤ P Ge ≤1.30) structures are clearly less stable ( E ≈−2.5 eV). This indicates that fully relaxed (aged) amorphous networks should not contain Ge H configurations. The energy distribution of Te atoms is simpler: twofold coordinated Te II are less stable than threefold Te III , with an energy difference of the order of 1.2 eV. The latter should thus be predominant in fully relaxed structures. 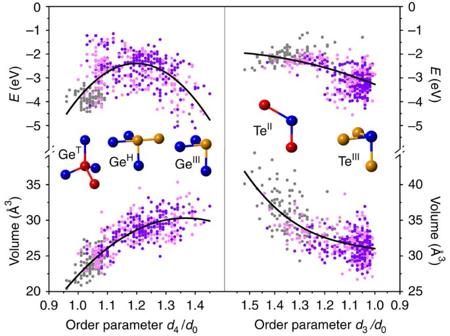Figure 3: Atomic energies and volume distributions in amorphous GeTe samples. The models are obtained from SiTe (grey), GeSe (light magenta) and SnTe (violet) parent structures by chemical substitution and annealing. Each point corresponds to an atom in the structures, whose environment is characterized by an order parameterPi, which can distinguish the different local structural motifs (seeSupplementary Note 3andSupplementary Fig. 4). Note the opposite direction of thex-axes in the two plots, so that the local structural relaxation proceeds from left to right in both. Black curves are parabolic fits to the data. Top panels: atomic energies. Bottom panels: atomic volumes calculated using a Voronoï tessellation analysis. The energy trends clearly indicate that GeIIIand TeIIIshould be predominant in relaxed amorphous structures. Figure 3: Atomic energies and volume distributions in amorphous GeTe samples. The models are obtained from SiTe (grey), GeSe (light magenta) and SnTe (violet) parent structures by chemical substitution and annealing. Each point corresponds to an atom in the structures, whose environment is characterized by an order parameter P i , which can distinguish the different local structural motifs (see Supplementary Note 3 and Supplementary Fig. 4 ). Note the opposite direction of the x -axes in the two plots, so that the local structural relaxation proceeds from left to right in both. Black curves are parabolic fits to the data. Top panels: atomic energies. Bottom panels: atomic volumes calculated using a Voronoï tessellation analysis. The energy trends clearly indicate that Ge III and Te III should be predominant in relaxed amorphous structures. Full size image The atomic volume distributions for Ge and Te show opposite trends. Tetrahedral Ge T have a smaller atomic volume than Ge III , while the associated Te II have a larger atomic volume than Te III . If we consider the two limiting cases, Ge T –Te II ( P Ge =1.0, P Te =1.5) versus Ge III –Te III ( P Ge =1.4, P Te =1.0), the volume differences are +7 Å 3 (Ge) and −8 Å 3 (Te), respectively. Altogether, the volume change for a GeTe mixture that accompanies the transition from Ge T –Te II to Ge III –Te III is thus negative. Neglecting the entropy contribution, the enthalpy ( U + PV ) is therefore always lower for Ge III and Te III (right side of the diagrams), in accordance with the maximal stability of the crystalline a-GeTe phase. At first sight, this seems to indicate that the local atomic order of the amorphous state is relaxing towards that of the crystal, as in the Zachariasen glass picture. However, a closer look at the electronic properties shows that, on the contrary, the amorphous state is relaxing away from the atomic arrangement of the crystal. Band gap widening The findings reported so far immediately raise the question how the properties of the amorphous state will change upon structural relaxation. From experiments, the optical band gap has been shown to widen on aging [43] . We have calculated the energy gap as a function of Ge T concentration (shown in Fig. 4a ) with GGA functionals, which yield a band gap of 0.41 eV for crystalline GeTe at the experimental density. For a-GeTe, it is more difficult to determine the conduction band minimum and the valence band maximum, due to the presence of (typically, strongly localized) defect states. To identify the latter states, we have carefully inspected the density of states near the Fermi energy and have determined their localization properties (see Supplementary Figs 5–8 ). The gap is only about 0.2±0.1 eV in the amorphous structures containing a majority of Ge T , whereas the structures that contain a small fraction of Ge T exhibit sizable gaps of the order of 0.5±0.1 eV. Therefore, an increase in the band gap is directly linked to a decrease in homopolar bonds and the concomitant disappearance of tetrahedrally bonded Ge atoms. Furthermore, this reduction is also accompanied by the disappearance of localized defect states in the band gap, as evidenced by the density of states plots shown in Fig. 4b . The contributions of the different species (Ge T , Ge H , Ge III , Te II and Te III ) to the band edge or in-gap states are displayed in Supplementary Fig. 5 , showing that the disappearance of the mid-gap states is due to the removal of homopolar bonds, whereas the band gap enlargement results from the enhancement of the Peierls distortion. 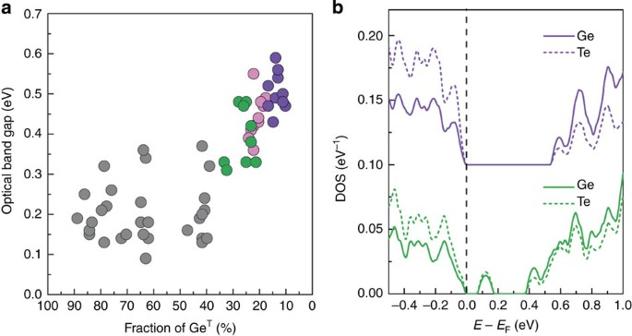Figure 4: Optical band gap and electronic density of states of various amorphous GeTe models. (a) Optical band gap of the relaxed amorphous GeTe models as a function of the fraction of tetrahedral Ge atoms (GeT) in the structure (same colour code asFig. 2). The optical gaps are calculated from the difference between the bottom of the valence band and the top of the conduction band. Some models possess localized defect states inside the gap IPR (seeSupplementary Figs 6-8). A reduction in the number of tetrahedrally coordinated Ge atoms leads to a larger optical band gap. (b) Density of states projected onto the orbitals of Ge atoms (solid curves) and Te atoms (dash-dot curves) for melt-quenched GeTe (green) and substituted a-SnTe (violet, shifted by 0.1 inyaxis). The melt-quenched model has a smaller band gap and possesses a (localized) mid-gap state. Figure 4: Optical band gap and electronic density of states of various amorphous GeTe models. ( a ) Optical band gap of the relaxed amorphous GeTe models as a function of the fraction of tetrahedral Ge atoms (Ge T ) in the structure (same colour code as Fig. 2 ). The optical gaps are calculated from the difference between the bottom of the valence band and the top of the conduction band. Some models possess localized defect states inside the gap IPR (see Supplementary Figs 6-8 ). A reduction in the number of tetrahedrally coordinated Ge atoms leads to a larger optical band gap. ( b ) Density of states projected onto the orbitals of Ge atoms (solid curves) and Te atoms (dash-dot curves) for melt-quenched GeTe (green) and substituted a-SnTe (violet, shifted by 0.1 in y axis). The melt-quenched model has a smaller band gap and possesses a (localized) mid-gap state. Full size image Photothermal deflection spectroscopy Subsequently, we have used PDS, which is very sensitive to small changes of band gap and low levels of absorption, to follow the temporal evolution of the electronic structure of an amorphous sample of GeTe ( Fig. 5a ). Our measurements of thick films enable the determination of the absorption coefficient over a large energy range. They confirm that, on aging, the band gap indeed increases, consistent with previous PDS [44] and ellipsometry data [43] . In addition, the PDS data in Fig. 5a reveal that the slope of the density of states close to the band gap (Urbach tail) does not change with aging. This behaviour is different from that of standard glasses like amorphous Si [45] , where aging is attributed to the decrease of the Urbach tails [46] . We have also computed absorption spectra using time-dependent DFT [47] , [48] in the adiabatic approximation and the vdW-DF2 functional ( Fig. 5b ). Consistent with the experimental data, aging is seen to lead to an increase in the band gap. Furthermore, the onset of the computed spectra shows strong absorption by defect states, in the case where a majority of Ge IV and Te II is present. These defect states, which are frequently located in the middle of the band gap, disappear on relaxation in favour of conduction states that are located just below or at the bottom of the conduction band. 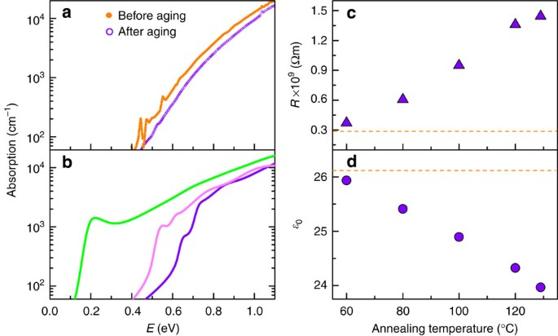Figure 5: Optical and dielectric properties of amorphous GeTe. (a) Experimental absorption measured by PDS. The orange and violet curves correspond to an a-GeTe 200-nm thick film measured before and after 1 h of aging (annealing) at 140 °C, respectively. The evolution of the curves is characteristic for the enlargement of the optical gap on aging. The Urbach energy, which characterizes the energy distribution of defect states at the band edges, does not change on annealing. (b) Absorption oscillator strength computed using time-dependent DFT for melt-quenched GeTe (green curve), and two models obtained from a-GeSe and a-SnTe by chemical substitution and annealing (light magenta and violet curves, respectively). Absorption peaks below∼0.6 eV correspond to defects, whereas the evolution of the curves between 0.6 and 1 eV matches the experimental increase in the optical gap. (c,d)The measurements of resistivity and epsilon staticɛ0of as-deposited amorphous GeTe on aging. The amorphous sample was heated at different annealing temperatures for 1 h before the measurements, taken at 120 K. The orange dashed lines mark the original values of resistivity andɛ0before aging (annealing). Aging is characterized by a significant decrease ofɛ0, which is very different from the value of the crystalline phase (∼180)49. Figure 5: Optical and dielectric properties of amorphous GeTe. ( a ) Experimental absorption measured by PDS. The orange and violet curves correspond to an a-GeTe 200-nm thick film measured before and after 1 h of aging (annealing) at 140 °C, respectively. The evolution of the curves is characteristic for the enlargement of the optical gap on aging. The Urbach energy, which characterizes the energy distribution of defect states at the band edges, does not change on annealing. ( b ) Absorption oscillator strength computed using time-dependent DFT for melt-quenched GeTe (green curve), and two models obtained from a-GeSe and a-SnTe by chemical substitution and annealing (light magenta and violet curves, respectively). Absorption peaks below ∼ 0.6 eV correspond to defects, whereas the evolution of the curves between 0.6 and 1 eV matches the experimental increase in the optical gap. ( c , d )The measurements of resistivity and epsilon static ɛ 0 of as-deposited amorphous GeTe on aging. The amorphous sample was heated at different annealing temperatures for 1 h before the measurements, taken at 120 K. The orange dashed lines mark the original values of resistivity and ɛ 0 before aging (annealing). Aging is characterized by a significant decrease of ɛ 0 , which is very different from the value of the crystalline phase ( ∼ 180) [49] . Full size image Dielectric properties To obtain further insights into the property changes that accompany aging, impedance spectroscopy experiments were performed on different amorphous GeTe samples. The samples were annealed for 1 h to successively higher temperatures. Subsequently, the resistance and the dielectric constant were both measured at 120 K. The aging process is clearly visible in the resistivity of the corresponding samples, which increases by almost a factor of 5, from 0.29 to 1.44 GΩm (see Fig. 5c ). Interesting enough, the aging process is also accompanied by a monotonous decrease of the static dielectric constant from 26.1 to 24 ( Fig. 5d ). For the crystalline state, the dielectric constant has been determined to be at least 180 by DFT calculations [49] . Hence, on aging, the dielectric properties of the amorphous phase become increasingly dissimilar from those of the crystal; the amorphous state thus ages away from the crystal. The significant decrease of the dielectric constant can be attributed to changes in bonding. According to ref. 50 , the dielectric constant ɛ 0 is computed using the formula, where the sum extends over all polar vibrational modes i , ω i being the frequency of the mode and the Born effective charge of the corresponding mode. Ω is the unit cell volume. We have calculated these quantities using linear response and the vdW-DF2 functional. The simulated dielectric constant ɛ 0 decreases from 34.1, the ‘young’ model (melt-quenched GeTe), down to 25.6, the more relaxed model (low-Ge T GeTe), which originates both from a reduction of ɛ ∞ from 22.6 to 16.7 and a decrease in the Born effective charges (see Supplementary Fig. 9 ). Indeed Ge H have on average a larger Z * than Ge III , their bonds being more polarizable. The disappearance of Ge T also leads to decreased ɛ 0 , but for a different reason: around these atoms, bonds are shorter and more covalent (thus less polarizable, yielding smaller Z *), but the gap is much smaller, causing the larger ɛ ∞. The more pronounced reduction of ɛ 0 in simulations ∼ 28% as compared with experiments ∼ 8%, can reasonably be attributed to the very likely large ‘age difference’ between the two AIMD models. While our method to generate amorphous models is representative of the various aging stages, it does not provide access to the time scale of the relaxation process. Nevertheless, it is interesting to note that the calculated ɛ 0 for the relaxed model is compatible with the measured ɛ 0 for the samples annealed at 60–80 °C (see Fig. 5d ). Peierls distortion To explain the decrease in Born effective charges, we have to clarify which atomic rearrangements characterize aging. Is this phenomenon solely related to the disappearance of homopolar Ge bonds and Ge T ? In fact, Fig. 2 already revealed that the process is more complex. It involves the transformation of Ge IV and Te II motifs to Ge III and Te III respectively, indicating that the local coordination becomes more crystal-like on aging. At the same time, the bond distances on aging become more dissimilar from the crystal. 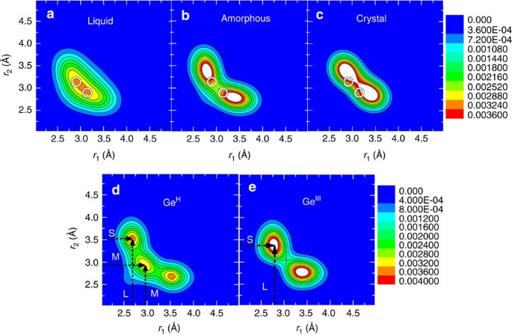Figure 6: Bond distributions around Ge in crystalline, liquid and relaxed amorphous GeTe. Plots have been obtained with vdW-DF2 functionals. The panels represent the angular-limited three-body correlation (ALTBC, normalized per atom), which expresses the probability of having a bond of lengthr1almost aligned with a bond of lengthr2(angular deviations smaller than 25°).r1andr2define the axes of the plots, which are symmetrical by nature. Top panels: (a) liquid phase atT=1,100 K, (b) relaxed glass obtained by substituting Sn with Ge in a-SnTe and (c) crystal. All systems are at the amorphous density. The white circles correspond to (r1,r2) in crystalline GeTe at the crystalline density. The plots show that the Peierls distortion ratio (r2/r1) in relaxed amorphous GeTe is larger than in the crystalline phase. Bottom panels: ALTBC plots for GeH(d) and GeIII(e). The plot for GeH(a high-energy defect, which disappears on aging) exhibits a broad distribution with three peaks corresponding to short–long (S-L) bonds and ‘medium-length’ bonds (M). On the contrary, the plot for the GeIIImotifs, which are predominant in the relaxed glass, displays two sharp, well-defined peaks corresponding to a genuine 3+3 Peierls distortion. Figure 6 shows the distribution of bond distances around Ge for the crystal, the liquid (at 1,100 K) and the relaxed amorphous state (the data for Te atoms are shown in the Supplementary Fig. 10 ). These plots clearly indicate that, in the relaxed glass, the Peierls distortion is more pronounced than in the other two states. In particular, average long/short bond distance ratios range from 1.20 (Ge) to 1.34 (Te) in the glass, whereas they are equal to 1.10 in the crystal. This property explains the larger band gap in relaxed amorphous GeTe with respect to the crystalline phase. Aging is not only characterized by the disappearance of Ge T defects, but also by the transition Ge H →Ge III , which brings about a more sharply defined Peierls-distorted network (see Fig. 6b and Supplementary Fig. 11 ). These two processes (a) lead to the suppression of conduction band tail and mid-gap defect states and (b) favour enhanced local distortions, contributing to the increase in the band gap. Figure 6: Bond distributions around Ge in crystalline, liquid and relaxed amorphous GeTe. Plots have been obtained with vdW-DF2 functionals. The panels represent the angular-limited three-body correlation (ALTBC, normalized per atom), which expresses the probability of having a bond of length r 1 almost aligned with a bond of length r 2 (angular deviations smaller than 25°). r 1 and r 2 define the axes of the plots, which are symmetrical by nature. Top panels: ( a ) liquid phase at T =1,100 K, ( b ) relaxed glass obtained by substituting Sn with Ge in a-SnTe and ( c ) crystal. All systems are at the amorphous density. The white circles correspond to ( r 1 , r 2 ) in crystalline GeTe at the crystalline density. The plots show that the Peierls distortion ratio ( r 2 / r 1 ) in relaxed amorphous GeTe is larger than in the crystalline phase. Bottom panels: ALTBC plots for Ge H ( d ) and Ge III ( e ). The plot for Ge H (a high-energy defect, which disappears on aging) exhibits a broad distribution with three peaks corresponding to short–long (S-L) bonds and ‘medium-length’ bonds (M). On the contrary, the plot for the Ge III motifs, which are predominant in the relaxed glass, displays two sharp, well-defined peaks corresponding to a genuine 3+3 Peierls distortion. Full size image Our results support the following qualitative model of aging in GeTe. The melt-quenched amorphous structures present a distribution of local environments. In particular, the fast-quenching process freezes in homopolar Ge-Ge bonds that form due to the low heat of formation of GeTe, and the concomitant tetrahedral structures. Other unfavourable atomic arrangements, which are frozen in on quenching, are fourfold coordinated Ge H atoms and twofold coordinated Te II atoms. Aging of the amorphous phase leads to the disappearance of these defects and to the increase in the number of threefold coordinated Ge and Te atoms. As a consequence, the fraction of Ge T decreases on aging, in line with the experimental evidences obtained by Mitrofanov et al. [51] , on the basis of XANES experiments. This structural evolution brings about a reduction in the number of mid-gap states. As a result, the chemical order and coordination numbers in the amorphous change towards those of the crystal. Yet, the atomic arrangement in amorphous Ge–Te is characterized by a significantly larger Peierls distortion. Qualitatively this scenario can be understood, since resonant bonding can only prevail for a moderate Peierls distortion. Hence, large local distortions become favourable in the amorphous state, where resonant bonding is absent [17] , [52] . As compared with other glassy systems, aging in GeTe displays peculiar features that set this system apart from the Zachariasen picture. Since the relaxed glass exhibits a larger Peierls distortion than the crystal, characteristic electronic properties of the amorphous state such as the band gap, electrical resistivity and dielectric constants drift away from those of the crystal during aging. This is very different from the behaviour of ordinary glasses, where structural relaxation leading to lower energy states is accompanied by an atomic rearrangement, which increasingly resembles the short-range order in the crystal. Our model is in agreement with all existing experimental data about aging of amorphous Ge x Sb y Te 1+ x + y alloys compounds. It not only provides an explanation for the technologically important resistivity drift phenomenon, but also emphasizes peculiarities of the amorphous phase of PCMs, beyond the already well-established unusual properties of the crystals. Since similar bonding patterns are present in Te-based amorphous PCMs, including the Sb 2 Te family, the microscopic mechanisms responsible for aging in amorphous GeTe should act similarly. Therefore, the evolution towards a strongly Peierls distorted network with coordination numbers similar to the crystal, but unlike chemical bonding and hence different bond lengths appears as a generic feature of the aging process in these systems. Computational details All the amorphous models contained 216 atoms and were generated with Perdew–Burke–Ernzerhof functionals based on the GGA [33] using QUICKSTEP [53] , a mixed Gaussian and plane-wave code implemented in the CP2K suite of programs [32] . The Kohn–Sham orbitals were expanded in a Gaussian basis set with triple/double-zeta plus polarization quality, whereas the electron density was expanded in plane waves with a cutoff of 300 Ry. Scalar-relativistic Goedecker–Teter–Hutter pseudopotentials [54] were employed. The Brillouin zone was sampled at the Gamma point only. The amorphous GeTe models produced under different chemical substitution conditions were further annealed with the vdW-DF2 functional [39] using PWSCF, a plane-wave code included in the Quantum Espresso package [55] . In this case, LDA norm-conserving pseudopotentials (Perdew and Zunger [56] ) were used with a 34 Ry cutoff energy for the kinetic energy. The molecular dynamics simulations were performed with a 3.84 fs time step and a Berendsen thermostat (relaxation time equal to 2.7 ps). The absorption spectra were computed using the turbo-Lanczos approach [48] with a total of 4,000 recursion coefficients. Amorphous models preparation is detailed in the Supplementary Method 1 . Photothermal deflection spectroscopy PDS is a highly sensitive technique to measure optical absorption (see Supplementary Method 2 ) [57] . PDS measurements on post-annealed and amorphous deposited phase-change films (sheet thickness d =200 nm) have been performed in cooperation with Reinhard Carius and Josef Klomfaß at the research center Jülich using a solid-state laser with a wavelength of λ =632 nm. Impedance spectroscopy Samples were prepared as a sandwich capacitor of 2 × 2 mm 2 with multilayers (Au/Cr/Ti/TiN/GeTe/TiN/Ti/Au/Cr/glass substrate). The thickness of GeTe, the electrode (Au/Cr) and the antidiffusion layer (TiN/Ti) are 463, 105 and 27 nm, respectively. The electrodes were prepared by thermal evaporation and all other layers by DC magnetron sputter deposition. The electrical impedance was measured via the Electrical Transport Option in a Quantum Design Physical Property Measurement System at the frequencies of 0.5–186 Hz from 4 to 150 K. Samples were annealed in the PPMS at different temperatures for one hour each with a ramp of 8 K.m −1 . Results are analysed with the equivalent circuit of a single paralleled RC model. How to cite this article: Raty, J. Y. et al. Aging mechanisms in amorphous phase-change materials. Nat. Commun. 6:7467 doi: 10.1038/ncomms8467 (2015).